Circadian regulation of intracellular G-protein signalling mediates intercellular synchrony and rhythmicity in the suprachiasmatic nucleus Synchronous oscillations of thousands of cellular clocks in the suprachiasmatic nucleus (SCN), the circadian centre, are coordinated by precisely timed cell–cell communication, the principle of which is largely unknown. Here we show that the amount of RGS16 (regulator of G protein signalling 16), a protein known to inactivate Gαi, increases at a selective circadian time to allow time-dependent activation of intracellular cyclic AMP signalling in the SCN. Gene ablation of Rgs16 leads to the loss of circadian production of cAMP and as a result lengthens circadian period of behavioural rhythm. The temporally precise regulation of the cAMP signal by clock-controlled RGS16 is needed for the dorsomedial SCN to maintain a normal phase-relationship to the ventrolateral SCN. Thus, RGS16-dependent temporal regulation of intracellular G protein signalling coordinates the intercellular synchrony of SCN pacemaker neurons and thereby defines the 24 h rhythm in behaviour. In mammals, the hypothalamic suprachiasmatic nucleus (SCN) is a central pacemaker, governing daily rhythms in behaviour and physiology [1] , [2] , [3] . Individual neurons in the SCN act as cell-autonomous oscillators, exhibiting circadian fluctuations of firing rate and gene expression [4] , [5] , [6] , [7] . We and others have recently shown that autonomous SCN neuronal oscillators maintain a high degree of synchrony with each other, so that they can generate coherent signals required for the circadian control of behaviour and physiology [6] , [7] , [8] , [9] , [10] . While individual SCN neurons share the same circadian period as a result of synchronization, the phases of their rhythms are strikingly diverse [6] . This observation reflects the reality that the SCN is an anatomically heterologous cellular assemblage, in which cohorts of differentially phased cellular clocks are deployed in a topographically specific manner [11] , [12] : neurons in the dorsomedial part of the SCN reach their daily peak in clock gene expression earlier in the day than those in the rest of the SCN. However, the mechanism by which dorsomedial SCN cells maintain their relatively advanced phasing, and to what extent this differential phasing influences the rhythms in behaviour have remained unknown. Much better understood is the molecular mechanism underlying cell-autonomous circadian oscillations. These rely on the opposing effects of transcriptional activators and repressors that generate negative feedback loops [13] , [14] , [15] . Briefly, the transcriptional activators CLOCK and BMAL1 drive transcription of Period ( Per1 and Per2 ) and Cryptochrome ( Cry1 and Cry2 ) genes via binding to E-box elements present in their promoters. Once the repressor proteins PER and CRY reach a critical concentration, they form complexes and repress their own expression by inhibiting the CLOCK/BMAL1 complexes. In addition to E-box elements, the promoter regions of Per genes contain D-boxes, through which the PAR bZip family of transcriptional activators (DBP, TEF and HLF) and the related repressor E4BP4 exert their opposing effects on the expression of target genes [16] , [17] , [18] , [19] , [20] . Finely controlled transcriptional regulation through the E-box and D-box motifs is thought to generate robust circadian expression of Per genes as well as a wide variety of clock-controlled genes [21] . Although cell-autonomous transcriptional regulation of clock genes could provide a common mechanism underlying the oscillations of individual cells, this does not explain the phasic differences between the neurons in the SCN. In this regard, it is important to note that the promoter region of Per1 gene contains a functional cyclic AMP-responsive element [22] , and that the extracellular signalling that activates cAMP pathway can acutely induce Per1 expression [23] . Because a light pulse given in the night time induces Per1 expression in the SCN, this pathway has long been considered crucial for light-dependent resetting of the phase of the molecular clock [24] , [25] , [26] . Yet, the cAMP-dependent control of Per1 may also have a role in coordinating circadian rhythms (phase-arrangement) of neurons in the SCN [14] . Supporting this hypothesis, the concentration of cAMP and transcriptional activity of the cAMP-responsive element in the SCN are both highly rhythmic even in constant darkness [27] , [28] , [29] . Moreover, pharmacological reduction in the rate of cAMP synthesis in the SCN lengthens the circadian period of the behavioural rhythm [29] , demonstrating a role of cAMP in the determination of the circadian period. RGS16 is a potential regulator of rhythmic cAMP synthesis in the SCN. Biochemically, RGS16 functions as a GTPase-accelerating protein for Gαi/o subtypes of G protein α subunits [30] , [31] , [32] . By promoting GTP hydrolysis, RGS16 terminates GTP-bound (thus activated) Gαi/o signalling. Microarray studies and the subsequent expression analyses revealed that the gene encoding RGS16 exhibits circadian variations in the levels of transcript in the SCN [33] , [34] , [35] , [36] . These data raise the possibility that Gαi/o-mediated cAMP signalling in the SCN is under circadian regulation via RGS16. Here we show that gene ablation of Rgs16 leads to the loss of circadian production of cAMP in the SCN, which results in a period lengthening of the locomotor activity rhythm. Extensive analysis of the intercellular phase-relationship within the SCN reveals that the RGS16-mediated daily activation of cAMP is necessary to accelerate the expression of Per1 in the dorsomedial cells. Our data therefore demonstrate that RGS16-mediated cAMP signalling defines the advanced phasing of dorsomedial cells, and as such, is a critical determinant for the period of circadian rhythms in behaviour. Gene expression profiles of the RGS family in the SCN It is known that pharmacological inhibition of Gαi/o activity with pertussis toxin hampers intercellular synchronization [37] and causes dampened rhythms of the entire SCN ( Supplementary Fig. S1 ) [37] . These observations prompted us to hypothesize that member(s) of the r egulator of G protein signalling (RGS) family might contribute to synchronized cellular oscillations in the SCN. We surveyed all known mouse Rgs genes for their expression in the SCN by using DNA microarray analysis ( Supplementary Fig. S2a ). Then, the genes highly expressed in the SCN were selected and further analysed with quantitative in situ hybridization to specify their histological distribution and circadian time (CT)-dependent expression profile ( Supplementary Fig. S2b ) [38] . This survey led us to notice that Rgs16 is the only RGS family member that displays marked SCN-specific expression particularly in the subjective daytime (see CT4 in Fig. 1a ; CT4 corresponds to 4 h after subjective onset of daytime under constant dark conditions). This expression profile, together with a prior work showing that RGS16 regulates Gαi/o activity [31] , [32] , raised the prospect that RGS16 contributes to SCN circadian clock physiology. 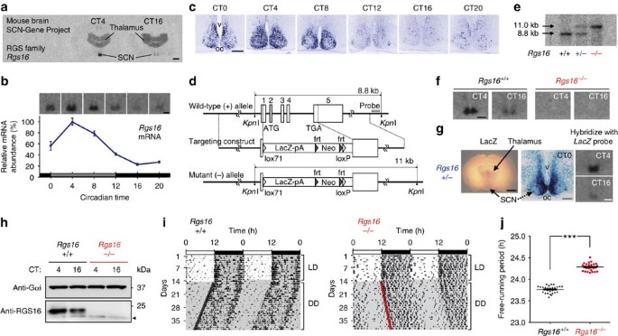Figure 1: RGS16 deficiency lengthens the circadian period of the locomotor activity rhythm. (a) Autoradiographs showing mouse coronal brain sections hybridized with anRgs16probe. CT4 and CT16 correspond respectively to 4 and 16 h after the subjective onset of daytime in DD. Bar, 1 mm. (b) Circadian expression ofRgs16in the SCN in DD. Relative RNA abundance was quantified with radioisotopicin situhybridization. Values means±s.e.m (n=5) with the peak value adjusted to 100. Representative autoradiographs at the indicated time points are shown on the top. Bar, 200 μm. (c) Digoxigeninin situhybridization showing the distribution ofRgs16-positive cells in the SCN. oc, optic chiasm; v, third ventricle. Bar, 100 μm. (d) Schematic representation of the mouseRgs16gene, targeting construct, and the mutant allele. Numbered boxes are the exons. The DNA probe used for southern blots is marked by a grey box. (e) Southern blot ofKpnI-digested DNA fromRgs16+/+,Rgs16+/–andRgs16−/−mice, WT (8.8 kb) and mutant (11 kb) allele. (f) Radioisotopicin situhybridization autoradiographs showing WT andRgs16−/−SCN. Bar, 200 μm. (g)Rgs16+/–coronal brain slice stained with X-gal (blue) with a magnified view of the SCN in a thin brain section at CT0. Autoradiographs show quantitativeLacZmRNAin situhybridization at CT4 and CT16. Scale bars: black, 1 mm, grey, 100 μm, white, 300 μm. (h) Western blots of RGS16 and Gαi in the SCN at CT4 and CT16. Arrowhead indicates a non-specific band. (i) Representative locomotor activity records of C57BL/6J-backcrossedRgs16+/+andRgs16−/−mice. Mice were housed in a 12L:12D light–dark cycle and then transferred to DD. Periods of darkness are indicated by grey backgrounds. The data are shown in double-plotted format. Each horizontal line represents 48 h; the second 24-h period is plotted to the right and below the first. The coloured lines delineate the phase of activity onset in DD. (j) Period-length distribution of C57BL/6J-backcrossedRgs16+/+andRgs16–/–mice. Free-running period measurements were based on a 14-day interval taken after 3 days of a DD regime and were executed with aχ2periodogram. Plotted are the period lengths of individual animals. Bars indicate mean±s.e.m. ***P<0.001, Student'st-test. Figure 1: RGS16 deficiency lengthens the circadian period of the locomotor activity rhythm. ( a ) Autoradiographs showing mouse coronal brain sections hybridized with an Rgs16 probe. CT4 and CT16 correspond respectively to 4 and 16 h after the subjective onset of daytime in DD. Bar, 1 mm. ( b ) Circadian expression of Rgs16 in the SCN in DD. Relative RNA abundance was quantified with radioisotopic in situ hybridization. Values means±s.e.m ( n =5) with the peak value adjusted to 100. Representative autoradiographs at the indicated time points are shown on the top. Bar, 200 μm. ( c ) Digoxigenin in situ hybridization showing the distribution of Rgs16 -positive cells in the SCN. oc, optic chiasm; v, third ventricle. Bar, 100 μm. ( d ) Schematic representation of the mouse Rgs16 gene, targeting construct, and the mutant allele. Numbered boxes are the exons. The DNA probe used for southern blots is marked by a grey box. ( e ) Southern blot of Kpn I-digested DNA from Rgs16 +/+ , Rgs16 +/– and Rgs16 −/− mice, WT (8.8 kb) and mutant (11 kb) allele. ( f ) Radioisotopic in situ hybridization autoradiographs showing WT and Rgs16 −/− SCN. Bar, 200 μm. ( g ) Rgs16 +/– coronal brain slice stained with X-gal (blue) with a magnified view of the SCN in a thin brain section at CT0. Autoradiographs show quantitative LacZ mRNA in situ hybridization at CT4 and CT16. Scale bars: black, 1 mm, grey, 100 μm, white, 300 μm. ( h ) Western blots of RGS16 and Gαi in the SCN at CT4 and CT16. Arrowhead indicates a non-specific band. ( i ) Representative locomotor activity records of C57BL/6J-backcrossed Rgs16 +/+ and Rgs16 −/− mice. Mice were housed in a 12L:12D light–dark cycle and then transferred to DD. Periods of darkness are indicated by grey backgrounds. The data are shown in double-plotted format. Each horizontal line represents 48 h; the second 24-h period is plotted to the right and below the first. The coloured lines delineate the phase of activity onset in DD. ( j ) Period-length distribution of C57BL/6J-backcrossed Rgs16 +/+ and Rgs16 –/– mice. Free-running period measurements were based on a 14-day interval taken after 3 days of a DD regime and were executed with a χ 2 periodogram. Plotted are the period lengths of individual animals. Bars indicate mean±s.e.m. *** P <0.001, Student's t -test. Full size image Cyclic expression of Rgs16 is driven by the circadian clock Time-dependent profiling revealed that Rgs16 exhibits overt circadian expression in the SCN ( Fig. 1b ), which persists even in constant darkness (DD) with a drastic increase of expression in the early subjective morning. Topographical analysis by digoxigenin in situ hybridization ( Fig. 1c ) further demonstrated that Rgs16 expression began to increase by subjective dawn (CT0) in the periventricular part of the dorsomedial SCN (a narrow but cell-dense area near the third ventricle). Thereafter, Rgs16 -positive staining spread widely across the SCN at CT4. At CT8, Rgs16 levels began to decrease in all SCN regions, and throughout the subjective night (that is, CT12–20) expression was limited to a few SCN cells. The spatiotemporal expression of Rgs16 resembles that of Per1 , a clock gene showing peak messenger RNA expression during the daytime in the SCN [11] , [12] . Similar to the Per1 promoter, the 5′-flanking genomic sequence of Rgs16 contains E-box and D-box cis -regulatory elements, thus allowing the circadian regulators CLOCK–BMAL1 and DBP to activate transcription. In a further parallel with Per1 , CRY1 and E4BP4 repressed CLOCK–BMAL1- and DBP-evoked Rgs16 expression, respectively ( Supplementary Figs. S3 and S4 ). Consistent with the promoter characteristics, in vivo circadian expression of Rgs16 was dramatically altered in the PAR bZip proteins-deficient mice ( Dbp −/− Tef −/− Hlf −/− ) [39] as well as Clock mutant and Cry1 −/− Cry2 −/− mice ( Supplementary Fig. S4f ). In Clock mutant mice, the early subjective day peak in Rgs16 expression was damped whereas in Cry1 −/− Cry2 −/− mice Rgs16 expression was high at both the subjective day and night time points. These data clearly demonstrate that expression of Rgs16 is under the control of the intracellular clock machinery. It is also noteworthy that the expression of Rgs16 was not light-inducible ( Supplementary Fig. S5 ). Thus, the internal clock seems to drive the morning expression of Rgs16 in the SCN. RGS16 deficiency lengthens the circadian period of behaviour To characterize the in vivo function of RGS16, we generated RGS16-deficient mice, in which a genomic region spanning whole coding sequence of Rgs16 was deleted and replaced with a lacZ reporter cassette ( Fig. 1d,e ). In situ hybridization analysis ( Fig. 1f ) confirmed the loss of the Rgs16 transcript in Rgs16 homozygous mutant ( Rgs16 −/− ) mice. β-galactosidase tissue staining ( Fig. 1g ) further corroborated gene targeting and replacement by LacZ : the spatio-temporal expression of the transgene reflected Rgs16 expression in the SCN. Moreover, we generated an antibody to RGS16 and performed immunoblot analysis with SCN extracts ( Fig. 1h ). As expected, the expression of RGS16 was not detected in Rgs16 −/− mice, whereas wild-type (WT) mice exhibited an increased expression of RGS16 protein in the subjective morning ( Fig. 1h ). We thus conclude that Rgs16 mutant mice are indeed RGS16-deficient. Behavioural analysis was performed with Rgs16 mutant mice that had been backcrossed to the C57BL/6J background over ten generations. We observed that the gene ablation of Rgs16 causes a lengthening of circadian period of the locomotor activity rhythm ( Fig. 1i ): under constant darkness, all Rgs16 −/− mice tested ( n =27) showed a free-running period longer than 24 h (circadian period (mean±s.e.m) determined with a χ 2 periodogram, 24.28±0.01 h). The phenotype of Rgs16 knockout sharply contrasts with that of Rgs16 +/+ control mice ( n =29), whose period is shorter than 24 h (23.76±0.01 h). The difference between the two genotypes is statistically significant ( Fig. 1j , P <0.001, Student's t -test) and does not depend on the way of measuring circadian period (periods determined with a linear regression line method: Rgs16 +/+ , 23.77±0.01 h; Rgs16 −/− , 24.31±0.01 h, P <0.001, Student's t -test), revealing that Rgs16 is a critical determinant of the behavioural rhythm period length. In contrast to the altered circadian periodicity under constant darkness, Rgs16 −/− mice displayed a normal 24 h rhythm when maintained in 12-h-light/12-h-dark cycle ( Fig. 1i ) and their resetting response to early and late night light pulses were indistinguishable from WT mice ( Supplementary Fig. S6 ). Thus, RGS16 is not necessary for light entrainment of the circadian clock. Rather, signalling through RGS16 comprises a pathway responsible for the maintenance of the normal circadian rhythm. RGS16 targets Gαi and regulates cAMP production in the SCN RGS16 is known to negatively regulate Gαi proteins, which downregulate cAMP production by inhibiting adenylate cyclase (AC) activity [31] , [32] . Double in situ hybridization revealed that both Gnai1 mRNA and Gnai2 mRNA (encoding Gαi1 and Gαi2, respectively) colocalize with Rgs16 in SCN neurons ( Fig. 2a ). Intriguingly, whereas the levels of Gαi1 and Gαi2 proteins were nearly constant throughout the day, the amount of RGS16 protein in the SCN showed overt circadian oscillation ( Fig. 2b ). Consistent with the GTPase-accelerating protein activity of RGS16, protein pull-down assays demonstrated that Gαi proteins in the SCN displayed an increased binding affinity for RGS16 when SCN extracts were treated with aluminium fluoride (AlF 4 − –GDP complex forms a transition state analogue of GTP hydrolysis) ( Fig. 2c ). Furthermore, immunoprecipitation of endogenous RGS16 protein at CT0 showed that the Gαi proteins coprecipitated with RGS16 from the protein extract of the WT SCN, but not from that of the Rgs16 −/− SCN ( Fig. 2d ). 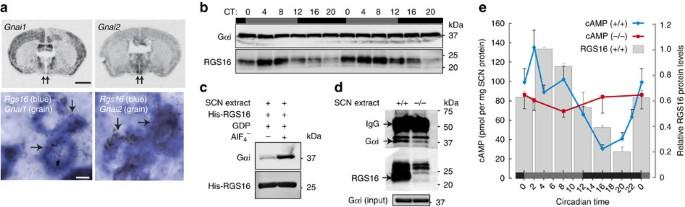Figure 2: RGS16 protein targets Gαi and regulates circadian production of cAMP in the SCN. (a) (Upper) Low-power film autoradiography showing the mouse coronal brain sectionsin situhybridized with radioisotopic probe forGnai1orGnai2. Arrows indicate the positions of the SCN. Bar, 2 mm. (Lower) High-power photomicrographs of the SCN doublein situhybridized with digoxigenin-labelled probe forRgs16(blue) and isotope-labelled probe forGnai1orGnai2(silver grains). Arrows indicate representative double-labelled cells. Bar, 5 μm. (b) Western blots analysing the temporal changes in the protein levels of RGS16 and Gαi in the WT mouse SCN. The animals kept in DD were killed at 4-h intervals across two circadian cycles (sampling times indicated at the top). The microdissected SCN extracts were probed with antibodies to RGS16 and Gαi. The Gαi antibody used recognizes both Gαi1 and Gαi2. (c) Increased binding affinity of RGS16 and Gαi in aluminium fluoride-treated SCN extracts. The microdissected SCN extract was incubated with His-tagged RGS16 protein in the presence of GDP with or without aluminium fluoride. Shown are Western blots of the proteins affinity purified with Ni-NTA beads. (d) Immunoprecipitation (IP) of endogenous Gαi with endogenous RGS16. The microdissected SCN extracts fromRgs16+/+orRgs16−/−mice at CT0 (input) were subjected to IP with RGS16 antibody. Shown are Western blots of the immunoprecipited RGS16 and Gαi (upper) and input Gαi (lower). (e) Circadian changes of cAMP content in the microdissected SCN fromRgs16+/+(blue) andRgs16−/−(red) mice (means±s.e.m,n=10, for each time point).P<0.01, CT2 (peak) versus CT16 (trough) inRgs16+/+mice. Such a temporal difference is not detected inRgs16−/−mice. To characterize more precisely the cAMP rhythm seen in WT mice, cAMP contents in the WT SCN were determined at shorter sampling intervals. The bar graph shows the levels of RGS16 protein in the SCN (means±range of variation) assessed from the results inbby densitometric analysis. Figure 2: RGS16 protein targets Gαi and regulates circadian production of cAMP in the SCN. ( a ) (Upper) Low-power film autoradiography showing the mouse coronal brain sections in situ hybridized with radioisotopic probe for Gnai1 or Gnai2 . Arrows indicate the positions of the SCN. Bar, 2 mm. (Lower) High-power photomicrographs of the SCN double in situ hybridized with digoxigenin-labelled probe for Rgs16 ( blue ) and isotope-labelled probe for Gnai1 or Gnai2 ( silver grains ). Arrows indicate representative double-labelled cells. Bar, 5 μm. ( b ) Western blots analysing the temporal changes in the protein levels of RGS16 and Gαi in the WT mouse SCN. The animals kept in DD were killed at 4-h intervals across two circadian cycles (sampling times indicated at the top). The microdissected SCN extracts were probed with antibodies to RGS16 and Gαi. The Gαi antibody used recognizes both Gαi1 and Gαi2. ( c ) Increased binding affinity of RGS16 and Gαi in aluminium fluoride-treated SCN extracts. The microdissected SCN extract was incubated with His-tagged RGS16 protein in the presence of GDP with or without aluminium fluoride. Shown are Western blots of the proteins affinity purified with Ni-NTA beads. ( d ) Immunoprecipitation (IP) of endogenous Gαi with endogenous RGS16. The microdissected SCN extracts from Rgs16 +/+ or Rgs16 −/− mice at CT0 (input) were subjected to IP with RGS16 antibody. Shown are Western blots of the immunoprecipited RGS16 and Gαi (upper) and input Gαi (lower). ( e ) Circadian changes of cAMP content in the microdissected SCN from Rgs16 +/+ (blue) and Rgs16 −/− (red) mice (means±s.e.m, n =10, for each time point). P <0.01, CT2 (peak) versus CT16 (trough) in Rgs16 +/+ mice. Such a temporal difference is not detected in Rgs16 −/− mice. To characterize more precisely the cAMP rhythm seen in WT mice, cAMP contents in the WT SCN were determined at shorter sampling intervals. The bar graph shows the levels of RGS16 protein in the SCN (means±range of variation) assessed from the results in b by densitometric analysis. Full size image Time-of-day specific inhibition of Gαi by RGS16 might affect circadian production of cAMP in the SCN, which has recently been proved crucial for the maintenance of robust circadian oscillations [29] . Consistent with this model, we found that cAMP concentrations in the WT SCN fluctuated in a circadian fashion, rising synchronously with the expression of RGS16 in the subjective morning ( Fig. 2e ). Furthermore, we observed that the circadian fluctuation of cAMP was abolished as a result of RGS16 deletion ( Fig. 2e ). Interestingly, in Rgs16 −/− mice, cAMP was maintained at intermediate levels throughout the day, implying that compensatory processes augment cAMP production. Hence, our data indicate that RGS16 is indispensable for conferring circadian rhythmicity (that is, time-of-day specificity) on the production of cAMP in the SCN. Delayed Per1 cycling in RGS16-deficient dorsomedial cells The Per1 gene is a central clock component that is linked to cAMP signalling through a cAMP-responsive element within its promoter region [22] ( Supplementary Fig. S3 ). Therefore, we examined the integrity of Per1 expression in the Rgs16 −/− SCN ( Fig. 3 ). Although circadian expression of Per1 in the mutant SCN was grossly normal, close inspection with digoxigenin in situ hybridization led us to identify a defect of Per1 expression in a small subset of cells located in the periventricular part of the dorsomedial SCN ( Fig. 3a ). Intriguingly, this region is anatomically characterized by a cluster of 'phase-leading' cells [11] , [12] in which Per1 mRNA levels peak at the beginning of the day, preceding the Per1 mRNA peak in ventral SCN cells. We observed that in Rgs16 −/− SCN, the rising phase of Per1 mRNA expression in the periventricular part of the dorsomedial SCN is significantly delayed, relative to that of WT SCN ( Fig. 3a and detailed profiles of Per1 expression in Supplementary Figs. S7 and S8 ). Thus, we speculated that cAMP signalling through RSG16 might be crucial for the phase-advanced expression of Per1 at dawn in the dorsomedially located phase-leading cells. 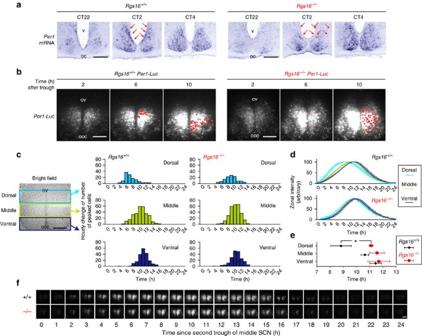Figure 3: RGS16 deficiency impairsPer1expression in dorsomedially located phase-leading cells. (a) Digoxigeninin situhybridization photomicrographs showing the topographical distributions ofPer1-positive cells in the SCN at CT22, CT2 and CT4. (b) Bioluminescent images of whole SCN slices fromPer1-luc-bearingRgs16+/+andRgs16−/−mice. The red spots on the right-side nucleus indicate the positions of the peaked cells at the indicated time point after the trough of the total SCN bioluminescence. (c) The range of peak times of randomly chosen cells from the subdivided dorsal (n=116, for each genotype), middle (n=281) and ventral (n=193) SCN zones of WT and mutant slices. For non-biased definition of the regions of interest, the SCN was divided into three regions with equal proportions along vertical axis (from the dorsal-most to the ventral-most). Thexaxis represents time (h) since 2nd trough of middle SCN luminescence. Note that the region selected as a dorsal zone encompasses the phase-leading cells. (d) The temporal changes in the levels of total luminescence from each zone (means±s.e.m (n=4); the peak and trough values were adjusted to 100 and 0, respectively). Two-way ANOVA with repeated measures identify a statistically significant interaction between zone and genotype (F(2, 18)=6.88,P<0.001). Bonferroni'spost hoctests reveal statistically significant difference between WT andRgs16−/−slices only in dorsal zone, but not in middle and ventral zones. (e) The average times of peaks (±s.d.) from subdivided dorsal, middle and ventral SCN zones of WT and mutant slices (n=4, for each genotype). *P< 0.001 (Bonferroni test). (f) Hourly images of the SCN slices fromRgs16+/+andRgs16−/−mice. See alsoSupplementary Movie 1. Scale bars in (a–f) are 100 μm. v, third ventricle; ov, original third ventricle; oc, optic chiasm; ooc, original optic chiasm. Figure 3: RGS16 deficiency impairs Per1 expression in dorsomedially located phase-leading cells. ( a ) Digoxigenin in situ hybridization photomicrographs showing the topographical distributions of Per1 -positive cells in the SCN at CT22, CT2 and CT4. ( b ) Bioluminescent images of whole SCN slices from Per1-luc -bearing Rgs16 +/+ and Rgs16 −/− mice. The red spots on the right-side nucleus indicate the positions of the peaked cells at the indicated time point after the trough of the total SCN bioluminescence. ( c ) The range of peak times of randomly chosen cells from the subdivided dorsal ( n =116, for each genotype), middle ( n =281) and ventral ( n =193) SCN zones of WT and mutant slices. For non-biased definition of the regions of interest, the SCN was divided into three regions with equal proportions along vertical axis (from the dorsal-most to the ventral-most). The x axis represents time (h) since 2nd trough of middle SCN luminescence. Note that the region selected as a dorsal zone encompasses the phase-leading cells. ( d ) The temporal changes in the levels of total luminescence from each zone (means±s.e.m ( n =4); the peak and trough values were adjusted to 100 and 0, respectively). Two-way ANOVA with repeated measures identify a statistically significant interaction between zone and genotype (F(2, 18)=6.88, P <0.001). Bonferroni's post hoc tests reveal statistically significant difference between WT and Rgs16 −/− slices only in dorsal zone, but not in middle and ventral zones. ( e ) The average times of peaks (±s.d.) from subdivided dorsal, middle and ventral SCN zones of WT and mutant slices ( n =4, for each genotype). * P < 0.001 (Bonferroni test). ( f ) Hourly images of the SCN slices from Rgs16 +/+ and Rgs16 −/− mice. See also Supplementary Movie 1 . Scale bars in ( a – f ) are 100 μm. v, third ventricle; ov, original third ventricle; oc, optic chiasm; ooc, original optic chiasm. Full size image To complement these observations, we analysed the Per1 expression profile in organotypic brain slices from Per1 promoter-luciferase ( Per1-luc ) transgenic mice [6] ( Fig. 3b-f ). Real-time bioluminescence imaging with high-resolution video microscopy [6] allows us to monitor the circadian dynamics of hundreds of individual neurons in morphologically preserved SCN slices [40] , where the luminescence driven by the Per1 promoter recapitulates the topographic- and time-dependent expression of Per1 mRNA ( Fig. 3b–f , Supplementary Fig. S9 and Supplementary Movie 1 , Per1-luc Rgs16 +/+ SCN). Thus, the phase-advanced oscillation, observable ex vivo in WT dorsomedial cells ( Fig. 3b–f ) is a property inherent to the SCN [6] . Taking advantage of this system, we examined Per1-luc rhythms in SCN slices from Rgs16 −/− mice ( Fig. 3b–f , Supplementary Fig. S9 and Supplementary Movie 1 , Per1-luc Rgs16 −/− SCN). In line with in vivo data from Rgs16 −/− mice, the luminescence of the Rgs16 −/− SCN slice was basically circadian, and its period was relatively long compared with that of WT slice (circadian period (h), mean±s.e.m., Rgs16 +/+ , 24.35±0.03; Rgs16 −/− , 24.82±0.07, n =6 for each genotype, P <0.05, t -test). Furthermore, when the phase differences across three SCN zones (dorsal, middle and ventral) were examined, the dorsal zone, which includes phase-leading cells, exhibited a delayed (relative to Rgs16 +/+ ) circadian oscillation, with a resultant phase close to that of the remaining zones ( Fig. 3d and Supplementary Fig. S9b ). Importantly, such alteration of dorsal rhythm was observed in all Rgs16 −/− SCN slice cultures tested, and statistical analysis revealed that the luminescence from the dorsal zone of the Rgs16 −/− SCN reached its peak at a time significantly later than that of the Rgs16 +/+ SCN ( Fig. 3e and Supplementary Fig. S9c ). Impaired cAMP signalling in RGS16-deficient dorsomedial cells The observations thus far indicate that dorsomedial SCN cells are the major (or sole) site where the RGS16-cAMP pathway could contribute to the rising phase of the Per1 mRNA. Consistent with this finding, we observed that the dawn expression of Per1 in the dorsomedial cells was unique in that it accompanied a strong induction of cFos ( Fig. 4a and Supplementary Fig. S10 ) [41] , [42] . as well as a simultaneous activation of extracellular signal-regulated kinase (ERK) ( Fig. 4b and Supplementary Fig. S10 ) [43] , [44] , [45] . Of note, both of these events were cAMP-dependent ( Fig. 4c–e ); hence, the pharmacological inhibition of cAMP synthesis in vivo with 9-(tetrahydro-2-furyl)-adenine (THFA, a noncompetitive AC inhibitor, which slows the rate of cAMP production but does not completely deplete cAMP [29] ) suppressed the dawn induction of cFos and phospho-ERK that otherwise appeared in the periventricular part of the dorsomedial SCN ( Fig. 4c–e and Supplementary Fig. S10 ). Thus, the activated cAMP pathway at dawn is a feature characterizing the phase-leading cells. 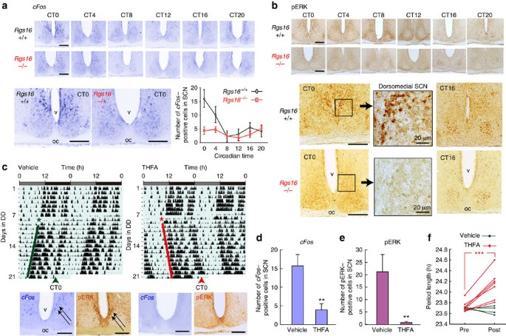Figure 4: RGS16 deficiency impairs cAMP-dependent induction ofcFosand ERK phosphorylation. (a) Digoxigeninin situhybridization photomicrographs showing the circadian profiles ofcFosexpression in the SCN ofRgs16+/+andRgs16−/−mice under DD conditions. The graph indicates the number ofcFos-positive cells (per section) across the circadian time (means±s.e.m,n=5). (b) Immunoreactivity to the pERK in the SCN ofRgs16+/+andRgs16−/−mice under DD conditions. (c) Representative locomotor activity records of WT mice under DD conditions before and after the surgery (asterisk) for the continuous infusion of THFA or vehicle (delivered to third ventricle just upper to the SCN via osmotic minipump). Arrowheads indicate the day on which the mice were killed at CT0 (estimated by the phase of the activity onset) for the analysis ofcFosand pERK expression in the SCN. Representative photomicrographs are shown below the locomotor activity records. Scale bars ina–care 100 μm unless otherwise noted. (d,e) The histograms showing the number (means±s.e.m) ofcFos- (d) or pERK- (e) positive cells in the SCN (per section) at CT0 after 14-days infusion of either THFA (n=6) or vehicle (n=6) in DD. **P<0.01,t-test, compared with vehicle treatments. (f) Pair-wised comparisons of behavioural periods before and after infusion of THFA (n=6) or vehicle (n=4). ***P<0.001, pairedt-test in THFA-treated mice. pERK, phosphorylated form of ERK. Figure 4: RGS16 deficiency impairs cAMP-dependent induction of cFos and ERK phosphorylation. ( a ) Digoxigenin in situ hybridization photomicrographs showing the circadian profiles of cFos expression in the SCN of Rgs16 +/+ and Rgs16 −/− mice under DD conditions. The graph indicates the number of cFos -positive cells (per section) across the circadian time (means±s.e.m, n =5). ( b ) Immunoreactivity to the pERK in the SCN of Rgs16 +/+ and Rgs16 −/− mice under DD conditions. ( c ) Representative locomotor activity records of WT mice under DD conditions before and after the surgery (asterisk) for the continuous infusion of THFA or vehicle (delivered to third ventricle just upper to the SCN via osmotic minipump). Arrowheads indicate the day on which the mice were killed at CT0 (estimated by the phase of the activity onset) for the analysis of cFos and pERK expression in the SCN. Representative photomicrographs are shown below the locomotor activity records. Scale bars in a – c are 100 μm unless otherwise noted. ( d , e ) The histograms showing the number (means±s.e.m) of cFos - ( d ) or pERK- ( e ) positive cells in the SCN (per section) at CT0 after 14-days infusion of either THFA ( n =6) or vehicle ( n =6) in DD. ** P <0.01, t -test, compared with vehicle treatments. ( f ) Pair-wised comparisons of behavioural periods before and after infusion of THFA ( n =6) or vehicle ( n =4). *** P <0.001, paired t -test in THFA-treated mice. pERK, phosphorylated form of ERK. Full size image Importantly, the dorsomedial cell-specific induction of cFos and ERK phosphorylation at dawn were both severely compromised by RGS16 deficiency ( Fig. 4a,b ), demonstrating that RGS16 determines the state of cAMP-dependent signalling in the phase-leading cells. We also observed that the animals treated with THFA phenocopied Rgs16 −/− mice ( Figs. 1i and 4c ), displaying a relatively long circadian locomotor activity rhythm ( Figs. 1j and 4f ). Thus, we concluded that cAMP signalling at dawn in the phase-leading cells depends on RGS16, and that the loss of RGS16-cAMP signalling causes a lengthening of the circadian period (or a constantly delayed phase) of the locomotor activity rhythm of mice. A critical issue for understanding SCN function is to identify how individual cellular clocks synchronize with a defined intercellular phase-relationship to broadcast coherent circadian signals to peripheral tissues and thereby coordinate physiology and behaviour. We previously showed that the dorsomedial SCN cells run ahead of the remaining cells, and that this differential phasing is an intrinsic property arising from the intercellular network of the SCN. However, the molecular mechanism underlying the phase-advanced oscillations of the dorsomedial cells and how they contribute to behavioural rhythms have remained unknown. In the present study, we have shown that the induction of dorsomedial Per1 expression at dawn is constantly accelerated by the circadian activation of intracellular cAMP signalling, which requires coordinated inhibition of Gαi by the clock-controlled RGS16 (see a schematic model in Fig. 5 ). Importantly, RGS16 deficiency, which delays dorsomedial Per1 expression, results in a period lengthening of behavioural rhythm. These data therefore reveal that the temporal regulation of intracellular G protein signalling that dictates the phasic arrangement within the SCN contributes to the determination of the circadian period of locomotor activity rhythm. 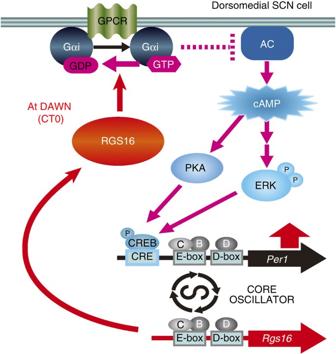Figure 5: Schematic model depicting a role of RGS16 in regulated cAMP signalling at dawn in the dorsomedial cells. Through allowing cAMP synthesis at dawn, RGS16 regulatesPer1expression in the dorsomedial phase-leading cells. B, BMAL1; C, CLOCK; CRE, cAMP responsive element; CREB, CRE-binding protein; D, DBP; P, phosphate; ERK, extracellular signal-regulated kinase; PKA, cAMP-dependent protein kinase. Figure 5: Schematic model depicting a role of RGS16 in regulated cAMP signalling at dawn in the dorsomedial cells. Through allowing cAMP synthesis at dawn, RGS16 regulates Per1 expression in the dorsomedial phase-leading cells. B, BMAL1; C, CLOCK; CRE, cAMP responsive element; CREB, CRE-binding protein; D, DBP; P, phosphate; ERK, extracellular signal-regulated kinase; PKA, cAMP-dependent protein kinase. Full size image We found that despite the disappearance of the cAMP rhythm, Rgs16 −/− mice still show Per1 oscillations in the SCN ( Fig. 3 ). This observation may be somewhat unexpected because pharmacological depletion of cAMP by an irreversible potent AC inhibitor (MDL-12,330A) constitutively reduces Per1 expression to basal levels [29] . It should be noted, however, that the concentrations of cAMP in the Rgs16 −/− SCN ( Fig. 2e ) and in THFA (a mild AC inhibitor)-treated cells [29] were not markedly reduced (kept at intermediate levels), and that under these conditions behavioural rhythms were sustainable, albeit with a relatively long circadian period ( Figs. 1i and 4c ) [14] . Consistent with this behavioural rhythm, the circadian fluctuations of Per1 in the Rgs16 −/− SCN were mostly unimpaired: rhythms in the vast majority of middle-to-ventral cells remained intact, and intriguingly, even in the dorsomedial cells, Per1 was still capable of oscillating, albeit with its peak phase significantly delayed due to RGS16 deficiency ( Fig. 3d,e ). Thus, the oscillations of Per1 in the SCN are not necessarily depending on the cAMP rhythm, but are rather self-sustainable, presumably due to transcriptional control through E-box and D-box, which might suffice to drive 'normal' (that is, non-phase-leading) Per1 expression. Our data therefore propose that the major role of the daily activation of cAMP in the SCN is to accelerate the expression of Per1 in the dorsomedial cells, thereby advancing the phases of these cells, relative to those of the cells in the middle-to-ventral SCN. RGS16 is an inhibitor of Gαi. How Gαi is activated in the SCN remains unknown. Gαi could be activated by extracellular or intracellular signals. One candidate, Dexras1, is a nonreceptor-associated activator for Gαi [46] . Interestingly, the gene encoding Dexras1 is highly and rhythmically expressed in the SCN, with a phase almost anti-phasic to that of Rgs16 , and mice lacking Dexras1 show abnormal desynchronization of the behavioural rhythm in constant light [47] . These results raise the prospect that the temporally segregated activation and inhibition of Gαi by Dexras1 and RGS16 might contribute to circadian control of Gαi. Besides Dexras1, Gαi-coupled GPCR signalling may also be involved. Defining which specific Gαi activators are required for SCN synchrony and how they act in concert with RGS16 will be our next challenge. It is also noteworthy that pharmacological (global) silencing of Gαi/o with pertussis toxin treatment could dampen SCN rhythm [37] , a phenotype differing from that of RGS16 deficiency. Thus, the mechanism(s) by which pertussis toxin affects SCN physiology remains unknown. We should also mention that RGS16 can target Gαq [30] . Given that in multiple cell types, Gαq-mediated Ca 2+ signalling interferes with cAMP production [48] , [49] , [50] , it will be worth testing whether Gαq signalling in the SCN is subject to the circadian regulation by RGS16 and how this potential pathway contributes to the altered cAMP signals in the RGS16-deficient SCN. In line with previous reports, we observed that the expression of cFos at dawn in the SCN is highly confined to the dorsomedial cells ( Fig. 4a ) [41] , [42] . This spatially limited activation of cFos cannot be explained by RGS16 distribution ( Fig. 1c ): cFos expression does not parallel the expression of Rgs16 in middle-to-ventral SCN regions, making it unlikely that RGS16 expression by itself suffices to drive cFos induction. Rather, given that the role of RGS16 is to inhibit Gαi and temporarily permit the production of cAMP in the SCN, it would be reasonable to speculate that RGS16 is necessary ( Fig. 4a ) but not sufficient to drive cAMP synthesis that triggers the expression of cFos in the dorsomedial cells. It is conceivable that the circadian regulation of cAMP is a multifactorial process involving not only Gαi but also Gαs. Along these lines, the vasoactive intestinal peptide, a neurotransmitter mediating cell–cell communication in the SCN, activates Gαs by acting through its cognate receptor VPAC 2 [8] , [9] , [51] . As it has been speculated that vasoactive intestinal peptide acts on the dorsomedial SCN [52] , further investigations aimed at deciphering the rules governing the precisely timed and topologically specific activation of Gαs and Gαi pathways in the SCN will be required to understand how cAMP synthesis in the SCN is controlled. Because the lengthened period of the Rgs16 −/− behavioural rhythm ( Fig. 1i,j ) is closely associated with the delayed phase of the periventricular part of the dorsomedial SCN ( Fig. 3a and Supplementary Figs. S7 and S8 ), we envisage that the functional changes in a small subset of neurons (for example, phase-leading cells) could alter the global timing property of the SCN. We observed that this prediction is mathematically feasible at least in a two-coupled cell-oscillator model that we constructed in silico ( Supplementary Fig. S11 ). The mathematical configuration used was based on a published model which hypothesizes a mutual coupling between the two oscillators [53] , [54] and was modified by introducing a term accounting for the dawn cAMP signal in a phase-leading cell (see Supplementary Methods for details). Under these conditions, the cell oscillating in silico with cAMP signalling at dawn runs ahead of the cell without cAMP signalling, and both cells exhibit the same circadian period (23.6 h) (see Supplementary Fig. S11 ). By contrast, once cAMP signalling was deleted from the phase-leading cell, then the two cells began to oscillate in phase with an elongated circadian period (24.4 h) ( Supplementary Fig. S11 ), a situation similar to what was observed for Rgs16 −/− mice under constant dark conditions. Thus, a modified two-coupled cell-oscillator model predicts the period lengthening by delayed circadian oscillation of phase-leading cells, whereas further elucidation of SCN network will be needed to faithfully recapitulate whole SCN function (see Supplementary Methods for detailed discussion). In conclusion, we provide evidence that RGS16, known as the regulator of intra cellular Gαi protein signalling, is a key component to establish the inter cellular phase-relationship of multi-phased SCN neurons. Mechanistically, RGS16 forms an integration point whereby the intracellular molecular clock exerts its effect on cAMP signalling ( Fig. 5 ). Through allowing cAMP synthesis at dawn, RGS16 in turn facilitates the phase-advanced expression of Per1 in the dorsomedial cells. Thus, our work adds a new layer of complexity to the rules that govern the intercellular synchrony of SCN neurons. We propose that signalling at the cell surface is not everything. Rather, the circadian time-dependent regulation of intracellular G protein signalling is also important to coordinate temporal and spatial order across the SCN. Furthermore, our work extends the role of RGS16 from cellular biology to behaviour. A major challenge in systems neuroscience is to integrate intra cellular molecular events with the inter cellular neural organization that gives rise to complex behavioural states. Using the SCN as a model, we show that the regulated intra cellular G-protein signalling that controls inter cellular synchrony across the SCN contributes to the determination of the period of daily rhythms in behaviour. Creation of Rgs16 knockout mice Rgs16 mutant mice (Acc. No. CDB0436K: http://www.cdb.riken.jp/arg/mutant%20mice%20list.html ) were generated according to our standard method [55] . The targeting vector was constructed using a bacterial artificial chromosome clone containing the mouse Rgs16 gene (RP24-576N23, BACPAC). We generated the 5′- and 3′-arms of Rgs16 ( Fig. 1d ) by PCR and cloned them into the corresponding sites of the DT-A/lox71/LacZ-pA/frt/PGK-Neo/frt/loxP/pA vector (the details of the vector are available in http://www.cdb.riken.go.jp/arg/cassette.html ). Gene targeting was carried out in TT2 cells [56] , an embryonic stem cell line established from F1 embryo between C57BL/6J female and CBA male (50% C57BL/6J, 50% CBA). Chimeric males were bred to wild type C57BL/6J females producing F1N0 progeny (75% C57BL/6J, 25% CBA). Germline transmission was verified by PCR as well as Southern blotting on tail DNA. F1N0 males were further backcrossed with C57BL/6J females to create F1N1 progeny (87.5% C57BL/6J). For behavioural analysis ( Fig. 1i,j ), we continued back-crossing up to F1N10 generation, which corresponds to 12 times backcrossing to the C57BL/6J background (>99.9% C57BL/6J) as the F1N0 mice with which we started backcrossing were already 75% C57BL/6J background. To conduct biochemical and histological analyses, we used F1N5 generation mice ( ∼ 99.2% C57BL/6J), the behavioural phenotypes of which are equivalent to those of F1N10 mice (free-running period (h) of F1N5 generation mice: Rgs16 +/+ , 23.58±0.03 (s.e.m. ), Rgs16 −/− , 24.35±0.03, n =6 for each genotype, P <0.01, t -test). We analysed littermate wild-type control mice having equivalent genetic backgrounds than the mutant mice. To this end, males and females from a specific generation (either F1N5 or F1N10 mice) were interbred to create a large colony. No difference in gross morphology or fertility was detected between the genotypes. Unless otherwise mentioned, in vivo comparative analyses of WT and mutant mice were conducted in DD. All the studies were approved by the animal experimentation committee of Kyoto University. Behavioural activity monitoring Single caged adult Rgs16 −/− mice and their wild-type littermates (male, 8–15 weeks old) were housed individually in light-tight, ventilated closets within a temperature- and humidity-controlled facility. The animals were entrained on a 12-h-light ( ∼ 200 lux fluorescent light)–12-h-dark cycle at least two weeks and then transferred to DD. Locomotor activity was detected with passive (pyroelectric) infra-red sensors (FA-05 F5B; Omron) [24] , [57] and the data obtained were analysed with Clocklab software (Actimetrics) developed on MatLab (Mathworks). Free-running period was determined with either a χ 2 periodogram or a linear regression line fit to the activity onsets. The data used for period measurements were based on animal behaviours in a 14-day interval taken 3 days after the start of DD condition. For the pulse-induced shift experiments, mice put in DD were exposed to a 15 min light pulse at either CT14 or CT22. Phase shifts (delay at CT14, advance at CT22) were quantified as the time difference between regression lines of activity onset before and after the light application. Microdissection of the mouse SCN The microdissection of the SCN was performed as described [27] with slight modifications. In brief, animals kept in DD were killed by cervical dislocation, and the eyes were removed under a safety red light. The brain was then isolated from the skull under room light and frozen immediately on dry ice. Coronal brain section (300 μm thick) containing the SCN was prepared using a cryostat microtome (CM3050S, Leica) and mounted on a silicon rubber stage at −17 °C. Under a magnifying glass, the bilateral SCN was punched out from the frozen section using a blunt 20-gauge syringe needle whose edge had been sharpened by filing. For the analysis of circadian expression of RGS16 and Gαi ( Fig. 2b ), the SCN punches ( n =3, for each time point) were pooled in Laemmli buffer, and the lysates were subjected to Western blot analysis with antibodies to RGS16 and Gαi. We generated rabbit polyclonal RGS16 antibody. The details of the antibodies used are available in Supplementary Methods . Pull down assay with His-tagged RGS16 RGS16 binding assay was performed as described [58] with slight modifications. In brief, the SCN punches ( n =5) were pooled in 300 μl of pull-down buffer (20 mM Na-HEPES, pH 8.0, 380 mM NaCl, 3 mM DTT, 6 mM MgCl 2 ) and homogenized by sonication at 4 °C (Bioruptor, COSMO BIO). The homogenate was divided into two aliquots and incubated with His-RGS16 protein (10 μg) in the presence of either GDP (10 μM) or GDP (10 μM) plus AlF 4 − (30 μM) for 30 min at 4 °C. The reaction mixtures were then treated with 1% cholate and centrifuged at 105,000 g (Optima MAX ultracentrifuge, Beckman). The detergent-soluble protein extracts were incubated with Ni2+-NTA agarose beads (Qiagen) for 15 min at 4 °C. Following three time washes with pull-down buffer supplemented with 20 mM imidazole (plus 10 μM GDP with or without 30 μM AlF 4 − ), the beads were boiled in Laemmli buffer. The protein complexes copurified with His-tagged RGS16 were analysed by Western blot. Immunoprecipitation with RGS16 antibody Immunoprecipitaion (IP) of RGS16 was performed with the SCN protein extracts from Rgs16 +/+ and Rgs16 −/− mice. The microdissected SCN punches ( n =5, for each pool) were homogenized in 300 μl of IP buffer (20 mM Na-HEPES, pH 8.0, 380 mM NaCl, 3 mM DTT, 6 mM MgCl 2 ,10 μM GDP and 30 μM AlF 4 − ) by sonication at 4 °C (Bioruptor, COSMO BIO). The homogenates were treated with 1% cholate and then centrifuged at 105,000 g (Optima MAX, Beckman). The detergent-soluble protein extracts were subjected to IP with RGS16 antibody and Protein A-Sepharose beads. After three time washes with IP buffer, the beads were boiled in Laemmli buffer. The proteins precipitated with RGS16 antibody were analysed by Western blot. cAMP measurement cAMP concentration was determined by enzyme immunoassay (EIA) using cAMP EIA kit (Cayman Chemical) according to the manufacturer's protocol. The microdissected SCN (one punch per assay) was collected in 300 μl of 0.1 N HCl solution and then sonicated at 4 °C (Bioruptor, COSMO BIO). The protein content was determined with BCA Protein Assay kit (Takara). Following centrifugation at 1,000 g for 10 min, the supernatant was diluted 1:2 with EIA buffer (Cayman Chemical). All SCN samples underwent acetylation before determination of cAMP level by EIA. We conducted the assays in duplicate, with measurement at l=405 nm on a plate reader (ARVO, Perkin-Elmer). Per1-luc SCN slice culture Per1-luc transgenic mice carry a firefly luciferase reporter gene linked to a 7.2 kb genomic DNA fragment covering the 5′ upstream region of the mouse Per1 gene [59] . Per1-luc - Rgs16 −/− mice were generated by crossing Per1-luc transgenic mice and Rgs16 −/− mice. The SCN slices were prepared according to our standard method [6] and kept at 35 °C in a sealed 35 mm petri dish with 1 ml of the culture medium containing 1 mM luciferin. The bioluminescence from the cultured SCN was measured with a highly sensitive cryogenic CCD camera (Spectra Video SV16KV/CT: Pixelvision) equipped with a microscope (Axiovert 135TV: Carl Zeiss). Observed data of images were filtered through a median filter to eliminate cosmic-ray-induced background noise. The luminescence was recorded every 20 min. Periods of SCN luminescence recordings were estimated using Fast Fourier Transform—Nonlinear Least Squares analysis [60] as part of the Biological Rhythms Analysis Software System (BRASS). For all SCN to be compared, identical segments of raw SCN luminescence values, starting from the first trough since the start of the measurement, and containing at least four complete cycles, were analysed. BRASS has been developed by Dr Brown PE and co-workers and is available from http://millar.bio.ed.ac.uk/Downloads.html . Intraventricular infusion of THFA THFA (Tocris) was continuously delivered to the SCN via osmotic pump as described [29] . In brief, the tip of the infusion cannula (Alzet, Brain Infusion Kit 2) was directed stereotaxically to the SCN and the osmotic pump (Alzet, pump model 1002) containing 100 mM THFA (118 μg/day, infused at 0.24 μl/h) was placed in a subcutaneous pouch by surgery under anaesthesia. We performed the surgery during the subjective daytime (CT8-10) when the phase of circadian clock is considered irresponsive to light. Following the surgery, animals were returned to their home cages and maintained in DD. Statistical analysis For the experiments in which three or more test groups were compared, we used one-way analysis of variance (ANOVA) with Bonferroni post-hoc test and evaluated the differences derived from genotypes and circadian time points tested. To assess the difference of circadian rhythm (phase) between the zones in Per1-luc SCN slices, we analysed the interaction between zone and circadian time with two-way repeated measures ANOVA, followed by Bonferroni's multiple comparison test. Additional methods Specific reagents and detailed methodology for DNA microarray analysis, in situ hybridization, X-gal staining, immunoblotting, immunohistochemistry and the antibodies used are all described in Supplementary Methods . Microarray data has been deposited in the Gene Expression Omnibus under accession code GSE28574. Accession codes: Microarray data has been deposited in the Gene Expression Omnibus under accession code GSE28574 . How to cite this article: Doi, M. et al . Circadian regulation of intracellular G-protein signalling mediates intercellular synchrony and rhythmicity in the suprachiasmatic nucleus. Nat. Commun. 2:327 doi: 10.1038/ncomms1316 (2011).